Real-time two-axis control of a spin qubit Optimal control of qubits requires the ability to adapt continuously to their ever-changing environment. We demonstrate a real-time control protocol for a two-electron singlet-triplet qubit with two fluctuating Hamiltonian parameters. Our approach leverages single-shot readout classification and dynamic waveform generation, allowing full Hamiltonian estimation to dynamically stabilize and optimize the qubit performance. Powered by a field-programmable gate array (FPGA), the quantum control electronics estimates the Overhauser field gradient between the two electrons in real time, enabling controlled Overhauser-driven spin rotations and thus bypassing the need for micromagnets or nuclear polarization protocols. It also estimates the exchange interaction between the two electrons and adjusts their detuning, resulting in extended coherence of Hadamard rotations when correcting for fluctuations of both qubit axes. Our study highlights the role of feedback in enhancing the performance and stability of quantum devices affected by quasistatic noise. Feedback is essential for stabilizing quantum devices and improving their performance. Real-time monitoring and control of quantum systems allows for precise manipulation of their quantum states [1] , [2] . In this way, it can help mitigate the effects of quantum decoherence and extend the lifetime of quantum systems for quantum computing and quantum sensing applications [3] , for example in superconducting qubits [4] , [5] , [6] , [7] , [8] , spins in diamond [9] , [10] , [11] , [12] , [13] , [14] , trapped atoms [15] , [16] , and other platforms [17] , [18] , [19] , [20] , [21] , [22] . Among the various quantum-information processing platforms, semiconductor spin qubits [23] , [24] are promising for quantum computing because of their long coherence times [25] and foundry compatibility [26] . Focusing on spin qubits hosted in gate-controlled quantum dots (QDs), two-qubit gate fidelities of 99.5% and single-qubit gate fidelities of 99.8% have recently been achieved in silicon [27] . In germanium, a four-qubit quantum processor based on hole spins enabled all-electric qubit logic and the generation of a four-qubit Greenberger-Horne-Zeilinger state [28] . In gallium arsenide, simultaneous coherent exchange rotations and four-qubit measurements in a 2 × 2 array of singlet-triplets were demonstrated without feedback, revealing site-specific fluctuations of nuclear spin polarizations [29] . In silicon, a six-qubit processor was operated with high fidelities enabling universal operation, reliable state preparation and measurement [30] . Achieving precise control of gated qubits can be challenging due to their sensitivity to environmental fluctuations, making feedback necessary to stabilize and optimize their performance. Because feedback-based corrections must be performed within the correlation time of the relevant fluctuations, real-time control is essential. Continuous feedback then allows to calibrate the qubit environment and to tune the qubit in real time to maintain high-fidelity gates and improved coherence, for instance by suppressing low-frequency noise and improving π -flip gate fidelity [31] . An active reset of a silicon spin qubit using feedback control was demonstrated based on quantum non-demolition readout [32] . Real-time operation of a charge sensor in a feedback loop [33] maintained the sensor sensitivity for fast charge sensing in a Si/SiGe double quantum dot, compensating for disturbances due to gate-voltage variation and 1/ f charge fluctuations. A quantum state with higher confidence than what is achievable through traditional thermal methods was initialized by real-time monitoring and negative-result measurements [34] . This study implements real-time two-axis control of a qubit with two fluctuating Hamiltonian parameters that couple to the qubit along different directions on its Bloch sphere. The protocol involves two key steps: first, rapid estimation of the instantaneous magnitude of one of the fluctuating fields (nuclear field gradient) effectively creates one qubit control axis. This control axis is then exploited to probe in real time the qubit frequency (Heisenberg exchange coupling) across different operating points (detuning voltages). Our procedure allows for counteracting fluctuations along both axes, resulting in an improved quality factor of coherent qubit rotations. Our protocol integrates a singlet-triplet (ST 0 ) spin qubit implemented in a gallium arsenide double quantum dot (DQD) [29] with Bayesian Hamiltonian estimation [35] , [36] , [37] , [38] , [39] . Specifically, an FPGA-powered quantum orchestration platform (OPX [40] ) repeatedly separates singlet-correlated electron pairs using voltage pulses and performs single-shot readout classifications to estimate on-the-fly the fluctuating nuclear field gradient within the double dot [41] . Knowledge of the field gradient in turn enables the OPX to coherently rotate the qubit between S and T 0 by arbitrary, user-defined target angles. Differently from previous works, we let the gradient freely fluctuate, without pumping the nuclear field [42] , and instead program the OPX to adjust the baseband control pulses accordingly. An adaptive second-axis estimation is performed to also probe the exchange interaction between the two electrons. This exchange interaction estimation scheme is not simply an independent repetition of the single-axis estimation protocol [35] , [36] , [37] , [38] , [39] : the design of the exchange-based free induction decay (FID) pulse sequence depends on the outcome of the first-axis estimation and needs to be computed on the fly. Finally, fluctuations along both axes are measured and corrected, enabling the stable coherent rotation of the qubit around a symmetric axis, essential for performing the Hadamard gate. Our work introduces a versatile method for enhancing coherent control and stability of spin qubits by harnessing low-frequency environmental fluctuations coupling to the system. As such, it is not limited to the operation of ST 0 qubits in GaAs. Our implementation of real-time reaction to fluctuating Hamiltonian parameters can find application in other materials and qubit encodings, as it is not necessarily limited to nuclear noise. Device and Bayesian estimation We use a top-gated GaAs DQD array [29] and tune up one of its ST 0 qubits using the gate electrodes shown in Fig. 1 c, at 200 mT in-plane magnetic field in a dilution refrigerator with a mixing-chamber plate below 30 mK. Radio-frequency reflectometry off the sensor dot’s ohmic contact distinguishes the relevant charge configurations of the DQD [43] . Fig. 1: A singlet-triplet (ST 0 ) qubit with two fluctuating control axes. a The dots' electrical detuning ε tunes from a regime of low qubit frequency, Ω L , to a regime of high frequency, Ω H . States outside the computational space are not plotted. b In the first (second) regime, the Overhauser gradient ∣ Δ B z ∣ (the exchange coupling J ) dominates the qubit frequency Ω L (Ω H ) and the polar angle φ of the qubit rotation axis. c SEM image of the GaAs device [29] , implementing a two-electron double quantum dot (black circles) next to its sensor dot (SD) for qubit readout. d J and Δ B z drive rotations of the qubit around two orthogonal axes, providing universal qubit control, as depicted in the Bloch sphere. e Uncontrolled fluctuations of the Larmor frequencies Ω L and Ω H , estimated in real time on the OPX and plotted with a 30 ms moving average. Full size image The qubit operates in the (1,1) and (0,2) charge configuration of the DQD. (Integers indicate the number of electrons in the left and right dot.) The electrical detuning ε quantifies the difference in the electrochemical potentials of the two dots, which in turn sets the qubit’s spectrum as shown in Fig. 1 a. We do not plot the fully spin-polarized triplet states, which are independent of ε and detuned in energy by the applied magnetic field. We define ε = 0 at the measurement point close to the interdot (1,1)-(0,2) transition, with negative ε in the (1,1) region. In the ST 0 basis, we model the time-dependent Hamiltonian by 
    ℋ(t)=J(ε (t)) σ_z/2+g^*_BΔB_z(t) σ_x/2,
 (1) which depends on the detuning ε that controls the exchange interaction between the two electrons, J ( ε ( t )), and the component of the Overhauser gradient parallel to the applied magnetic field between the two dots, Δ B z ( t ). σ i are the Pauli operators, g * is the effective g-factor, and μ B is the Bohr magneton. In the following, we drop the time dependence of the Hamiltonian parameters for ease of notation. On the Bloch sphere of the qubit (Fig. 1 d), eigenstates of the exchange interaction, \(\left\vert {{{{{{{\rm{S}}}}}}}}\right\rangle\) and \(\left\vert {{{{{{{{\rm{T}}}}}}}}}_{0}\right\rangle\) , are oriented along Z , while Δ B z enables rotations along X . The qubit is manipulated by voltage pulses applied to the plunger gates of the DQD, and measured near the interdot (1,1)-(0,2) transition by projecting the unknown spin state of (1,1) onto either the (1,1) charge state ( \(\left\vert {{{{{{{{\rm{T}}}}}}}}}_{0}\right\rangle\) ) or the (0,2) charge state ( \(\left\vert {{{{{{{\rm{S}}}}}}}}\right\rangle\) ). Each single-shot readout of the DQD charge configuration involves generation, demodulation, and thresholding of a few-microsecond-long radio-frequency burst on the OPX (see Supplementary Fig. 1) . The OPX allows for real-time calculation of the qubit Larmor frequency \({{\Omega }}(\varepsilon )=\scriptstyle\sqrt{{{\Delta }}{B}_{z}^{2}+J{(\varepsilon )}^{2}}\) at different detunings, based on real-time estimates of Δ B z and J ( ε ). Inspecting the exchange coupling in a simplified Fermi-Hubbard hopping model [23] and inserting J ( ε ) into Eq. ( 1 ) suggests two physically distinct regimes [Fig. 1 b]: At low detuning, in the (1,1) charge state configuration, the Overhauser gradient dominates the qubit dynamics. In this regime, the qubit frequency reads \({{{\Omega }}}_{{{{{{{{\rm{L}}}}}}}}}\equiv \scriptstyle\sqrt{{{\Delta }}{B}_{z}^{2}+{J}_{{{{{{{{\rm{res}}}}}}}}}^{2}}\) , where we have added a small phenomenological term \({J}_{{{{{{{{\rm{res}}}}}}}}}\) to account for a constant residual exchange between the two electrons at low detuning. Such a term may become relevant when precise knowledge of Δ B z is required, for example for the Hadamard protocol at the end of this study. At high detuning, close to the (1,1)–(0,2) interdot charge transition, exchange interaction between the two electrons dominates, and the qubit frequency becomes \({{{\Omega }}}_{{{{{{{{\rm{H}}}}}}}}}(\varepsilon )\equiv \scriptstyle\sqrt{{{\Delta }}{B}_{z}^{2}+J{(\varepsilon )}^{2}}\) . As shown in Fig. 1 b, the detuning affects both the Larmor frequency Ω and the polar angle φ of the qubit rotation axis \(\hat{{{{{{{{\boldsymbol{\omega }}}}}}}}}\) , with φ approaching 0 in the limit J ( ε ) ≫ Δ B z and π /2 if J ( ε ) ≪ Δ B z . Without the possibility of turning off either J or Δ B z , the rotation axes of the singlet-triplet qubit are tilted, meaning that pure X - and Z -rotations are unavailable. In their absence, the estimation of the qubit frequency at different operating points is crucial for navigating the whole Bloch sphere of the qubit. 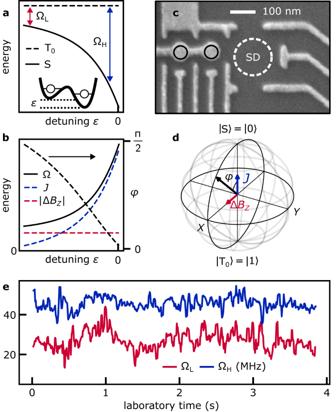Fig. 1: A singlet-triplet (ST0) qubit with two fluctuating control axes. aThe dots' electrical detuningεtunes from a regime of low qubit frequency, ΩL, to a regime of high frequency, ΩH. States outside the computational space are not plotted.bIn the first (second) regime, the Overhauser gradient∣ΔBz∣(the exchange couplingJ) dominates the qubit frequency ΩL(ΩH) and the polar angleφof the qubit rotation axis.cSEM image of the GaAs device29, implementing a two-electron double quantum dot (black circles) next to its sensor dot (SD) for qubit readout.dJand ΔBzdrive rotations of the qubit around two orthogonal axes, providing universal qubit control, as depicted in the Bloch sphere.eUncontrolled fluctuations of the Larmor frequencies ΩLand ΩH, estimated in real time on the OPX and plotted with a 30 ms moving average. Figure 1 e tracks Larmor frequencies Ω H and Ω L , both fluctuating over tens of MHz over a period of several seconds, using a real-time protocol as explained later. The presence of low-frequency variations in time traces of Ω H and Ω L suggests that qubit coherence can be extended by monitoring these uncontrolled fluctuations in real time and appropriately compensating qubit manipulation pulses on-the-fly. To estimate the frequency of the fluctuating Hamiltonian parameters on the OPX, we employ a Bayesian estimation approach based on a series of free-induction-decay experiments [35] . Using m i to represent the outcome ( \(| {{{{{{{\rm{S}}}}}}}}\rangle\) or \(| {{{{{{{{\rm{T}}}}}}}}}_{0}\rangle\) ) of the i -th measurement after an evolution time t i , the conditional probability P ( m i ∣ Ω) is defined as the probability of obtaining m i given a value of Ω: 
    P(m_i| Ω)=1/2[1+r_i(α+βcos(2πΩt_i))],
 (2) where r i takes a value of 1 ( − 1) if \({m}_{i}=\vert {{{{{{{\rm{S}}}}}}}}\rangle\) ( \(\left\vert {{{{{{{{\rm{T}}}}}}}}}_{0}\right\rangle\) ), and α and β are determined based on the measurement error and axis of rotation on the Bloch sphere. Applying Bayes’ rule to estimate Ω based on the observed measurements m N , … m 1 , which are assumed to be independent of each other, yields the posterior probability distribution \(P\left({{\Omega }}\,| {m}_{N},\ldots {m}_{1}\right)\) in terms of a prior uniform distribution \({P}_{0}\left({{\Omega }}\right)\) and a normalization constant \({{{{{{{\mathcal{N}}}}}}}}\) : 
    P(Ω | m_N,…m_1)=	 P_0(Ω)𝒩
    ×∏_i=1^N[1+r_i(α+βcos(2πΩt_i))]. (3) Based on previous works [35] , [38] , [39] , we fix α = 0.25 and β = ±0.5, with the latter value positive when estimating Ω L and negative when estimating Ω H . The expectation value 〈Ω〉, calculated over the posterior distribution after all N measurements, is then taken as the final estimate of Ω. Controlled Overhauser gradient driven rotations We first implement qubit control using one randomly fluctuating Hamiltonian parameter, through rapid Bayesian estimation of Ω L and demonstration of controlled rotations of a ST 0 qubit driven by the prevailing Overhauser gradient. Notably, this allows coherent control without a micromagnet [44] , [45] or nuclear spin pumping [42] . Ω L is estimated from the pulse sequence shown in Fig. 2 a: for each repetition a singlet pair is initialized in (0,2) and subsequently detuned deep in the (1, 1) region ( ε L ≈ − 40 mV) for N = 101 linearly spaced separation times t i up to 100 ns. After each separation, the qubit state, \(\left\vert {{{{{{{\rm{S}}}}}}}}\right\rangle\) or \(\left\vert {{{{{{{{\rm{T}}}}}}}}}_{0}\right\rangle\) , is assigned by thresholding the demodulated reflectometry signal V rf near the (1,1)-(0,2) interdot transition and updating the Bayesian probability distribution of Ω L according to the outcome of the measurement. After measurement m N , the initially uniform distribution has narrowed [inset of Fig. 2 b, with white and black indicating low and high probability], allowing the extraction of 〈Ω L 〉 as the estimate for Ω L . For illustrative purposes, we plot in Fig. 2 a the N single-shot measurements m i for 10,000 repetitions of this protocol, which span a period of about 20 s, and in Fig. 2 b the associated probability distribution P (Ω L ) of each repetition. The quality of the estimation seems to be lower around a laboratory time of 6 seconds, coinciding with a reduced visibility of the oscillations in panel 2 a. We attribute this to an enhanced relaxation of the triplet state during readout due to the relatively high ∣ Δ B z ∣ gradient during those repetitions [46] . The visibility could be improved by a latched or shelved read-out [47] , [48] or energy-selective tunneling-based readout [38] . Fig. 2: Controlled Overhauser gradient driven rotations of a ST 0 qubit by real-time Bayesian estimation. One loop (solid arrows) represents one repetition of the protocol. a For each repetition, the OPX estimates Ω L by separating a singlet pair for N linearly spaced probe times t i and updating the Bayesian estimate (BE) distribution after each measurement, as shown in the inset of b for one representative repetition. For illustrative purposes, each single-shot measurements m i is plotted as a white/black pixel, here for N = 101 Ω L probe cycles, and the fraction of singlet outcomes in each column is shown as a red dot. b Probability distribution P (Ω L ) after completion of each repetition in a. Extraction of the expected value 〈Ω L 〉 from each row completes Ω L estimation. c For each repetition, unless 〈Ω L 〉 falls below a user-defined minimum (here 50 MHz), the OPX adjusts the separation times \({\tilde{t}}_{j}\) , using its real-time knowledge of 〈Ω L 〉, to rotate the qubit by user-defined target angles \({\theta }_{j}={\tilde{t}}_{j}\,\langle {{{\Omega }}}_{{{{{{{{\rm{L}}}}}}}}}\rangle\) . d To illustrate the increased coherence of Overhauser gradient driven rotations, we task the OPX to perform M = 80 evenly spaced θ j rotations. Single-shot measurements m j are plotted as white/black pixels, and the fraction of singlet outcomes in each column is shown as a red dot. Full size image Even though the rotation speed around \({\hat{{{{{{{{\boldsymbol{\omega }}}}}}}}}}_{{{{{{{{\rm{L}}}}}}}}}\) at low detuning is randomly fluctuating in time, knowledge of 〈Ω L 〉 allows controlled rotations by user-defined target angles. To show this, we task the OPX in Fig. 2 d to adjust the separation times \({\tilde{t}}_{j}\) in the pulse sequence to rotate the qubit by M = 80 different angles \({\theta }_{j}={\tilde{t}}_{j}\,\langle {{{\Omega }}}_{{{{{{{{\rm{L}}}}}}}}}\rangle\) between 0 and 8 π . In our notation, the tilde in a symbol \(\tilde{x}\) indicates that the waveform parameter x is computed dynamically on the OPX. To reduce the FPGA memory required for preparing waveforms with nanosecond resolution, we perform controlled rotations only if the expected Ω L is larger than an arbitrarily chosen minimum of 50 MHz. (The associated IF statement and waveform compilation then takes about 40 μs on the FPGA.) This reduces the number of precomputed waveforms needed for the execution of pulses with nanosecond-scale granularity, for which we use the OPX baked waveforms capability. Accordingly, the number of rows in Fig. 2 d (1450) is smaller than in panel a, and we only label a few selected rows with their repetition number. To show the increased rotation-angle coherence of controlled ∣ Δ B z ∣ -driven rotations, we plot the average of all 1450 repetitions of Fig. 2 d and compare the associated quality factor, Q ≳ 7, with that of uncontrolled oscillations, Q ~ 1 (we define the quality factor as the number of oscillations until the amplitude is 1/e of its original value). The average of the uncontrolled S-T 0 oscillations in Fig. 2 a can be fit by a decay with Gaussian envelope (solid line), yielding an inhomogeneous dephasing time \({T}_{2}^{*}\,\approx\, 30\,{{{{{{{\rm{ns}}}}}}}}\) typical for ST 0 qubits in GaAs [49] . We associate the relatively smaller amplitude of stabilized qubit oscillations with the low-visibility region around 6 seconds in Fig. 2 d, discussed earlier. Excluding such regions by post selection increases the visibility and quality factor of oscillations (see Supplementary Fig. 4 ). Overall, the results presented in this section exemplify how adaptive baseband control pulses can operate a qubit reliably, out of slowly fluctuating environments. 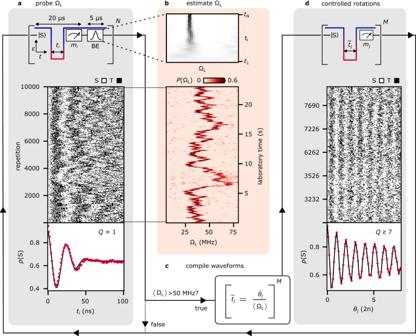Fig. 2: Controlled Overhauser gradient driven rotations of a ST0qubit by real-time Bayesian estimation. One loop (solid arrows) represents one repetition of the protocol.aFor each repetition, the OPX estimates ΩLby separating a singlet pair forNlinearly spaced probe timestiand updating the Bayesian estimate (BE) distribution after each measurement, as shown in the inset of b for one representative repetition. For illustrative purposes, each single-shot measurementsmiis plotted as a white/black pixel, here forN= 101 ΩLprobe cycles, and the fraction of singlet outcomes in each column is shown as a red dot.bProbability distributionP(ΩL) after completion of each repetition in a. Extraction of the expected value 〈ΩL〉 from each row completes ΩLestimation.cFor each repetition, unless 〈ΩL〉 falls below a user-defined minimum (here 50 MHz), the OPX adjusts the separation times\({\tilde{t}}_{j}\), using its real-time knowledge of 〈ΩL〉, to rotate the qubit by user-defined target angles\({\theta }_{j}={\tilde{t}}_{j}\,\langle {{{\Omega }}}_{{{{{{{{\rm{L}}}}}}}}}\rangle\).dTo illustrate the increased coherence of Overhauser gradient driven rotations, we task the OPX to performM= 80 evenly spacedθjrotations. Single-shot measurementsmjare plotted as white/black pixels, and the fraction of singlet outcomes in each column is shown as a red dot. Real-time two-axis estimation In addition to nuclear spin noise, ST 0 qubits are exposed to electrical noise in their environment, which affects the qubit splitting in particular at higher detunings. 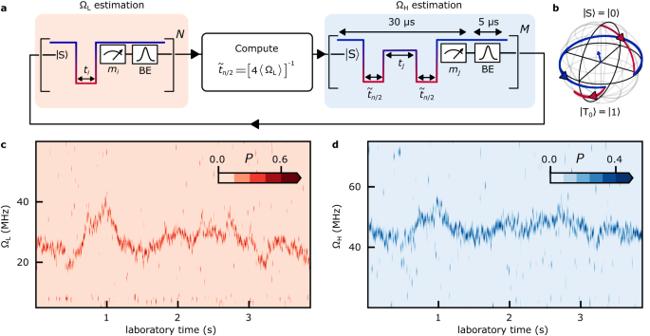Fig. 3: Real-time Bayesian estimation of two control axes. aOne repetition of the two-axis estimation protocol. After estimating ΩLfromN= 101tiprobe cycles (Fig.2a), the OPX computes on-the-fly the pulse duration\({\tilde{t}}_{\pi /2}\)required to initialize the qubit near the equator of the Bloch sphere by a diabatic ΩL(π/2) pulse. After the ΩL(π/2) pulse, the qubit evolves for timetjunder exchange interaction before another ΩL(π/2) pulse initiates readout. After each single-shot measurementmj, the OPX updates the BE distribution of ΩH. Similar totiin the ΩLestimation,tjis spaced evenly between 0 and 100 ns acrossM= 101 exchange probe cycles.bQubit evolution on the Bloch sphere during one exchange probe cycle.cEach column plotsP(ΩL) after completion of the ΩLestimation in each protocol repetition.dEach column plotsP(ΩH) after completion of the ΩHestimation in each protocol repetition. It is therefore important to examine and mitigate low-frequency noise at different operating points of the qubit. In the previous section, the qubit frequency Ω L was estimated entirely at low detuning where the Overhauser field gradient dominates over the exchange interaction. In order to probe and stabilize also the second control axis, namely J -driven rotations corresponding to small φ in Fig. 1 d, we probe the qubit frequency Ω H at higher detunings, using a similar protocol with a modified qubit initialization. Free evolution of the initial state \(\left\vert {{{{{{{\rm{S}}}}}}}}\right\rangle\) around \({\hat{{{{{{{{\boldsymbol{\omega }}}}}}}}}}_{{{{{{{{\rm{L}}}}}}}}}\) would result in low-visibility exchange-driven oscillations because of the low value of φ . To circumvent this problem, we precede the Ω H estimation by one repetition of Ω L estimation, as shown in Fig. 3 a. This way, real-time knowledge of 〈Ω L 〉 allows the initial state \(\left\vert {{{{{{{\rm{S}}}}}}}}\right\rangle\) to be rotated to a state near the equator of the Bloch sphere, before it evolves freely for probing Ω H . This rotation is implemented by a diabatic detuning pulse from (0,2) to ε L (diabatic compared to the interdot tunnel coupling) for time \({\tilde{t}}_{\pi /2}\) , corresponding to a rotation of the qubit around \({\hat{{{{{{{{\boldsymbol{\omega }}}}}}}}}}_{{{{{{{{\rm{L}}}}}}}}}\) by an angle \({{{\Omega }}}_{{{{{{{{\rm{L}}}}}}}}}{\tilde{t}}_{\pi /2}=\pi /2\) . After evolution for time t j under finite exchange, another π /2 rotation around \({\hat{{{{{{{{\boldsymbol{\omega }}}}}}}}}}_{{{{{{{{\rm{L}}}}}}}}}\) rotates the qubit to achieve a high readout contrast in the ST 0 basis, as illustrated on the Bloch sphere in Fig. 3 b. Fig. 3: Real-time Bayesian estimation of two control axes. a One repetition of the two-axis estimation protocol. After estimating Ω L from N = 101 t i probe cycles (Fig. 2 a), the OPX computes on-the-fly the pulse duration \({\tilde{t}}_{\pi /2}\) required to initialize the qubit near the equator of the Bloch sphere by a diabatic Ω L ( π /2) pulse. After the Ω L ( π /2) pulse, the qubit evolves for time t j under exchange interaction before another Ω L ( π /2) pulse initiates readout. After each single-shot measurement m j , the OPX updates the BE distribution of Ω H . Similar to t i in the Ω L estimation, t j is spaced evenly between 0 and 100 ns across M = 101 exchange probe cycles. b Qubit evolution on the Bloch sphere during one exchange probe cycle. c Each column plots P (Ω L ) after completion of the Ω L estimation in each protocol repetition. d Each column plots P (Ω H ) after completion of the Ω H estimation in each protocol repetition. Full size image As a side note, we mention that in the absence of knowledge of the Overhauser field gradient, the qubit would traditionally be initialized near the equator by adiabatically reducing detuning from (0,2) to the (1,1) charge configuration, and a reverse ramp for readout. Such adiabatic ramps usually last several microseconds each, while our \({\tilde{t}}_{\pi /2}\) pulses typically take less than 10 ns, thereby significantly shortening each probe cycle. For the estimate of Ω H , the Bayesian probability distribution of Ω H is updated after each of the M = 101 single-shot measurement m j , each corresponding to a separation time t j that is evenly stepped from 0 to 100 ns. The Bayesian probability distributions of both Ω L and Ω H are shown in Fig. 3 c and d, respectively, with the latter being conditioned on 20 MHz < 〈Ω L 〉 < 40 MHz to reduce the required FPGA memory. This section demonstrated a real-time baseband control protocol that enables manipulation of a spin qubit on the entire Bloch sphere. Controlled exchange-driven rotations Using Bayesian inference to estimate control axes in real-time offers new possibilities for studying and mitigating qubit noise at all detunings. 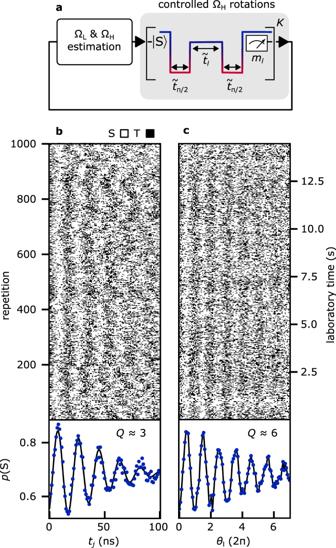Fig. 4: Real-time-controlled exchange-driven qubit rotations. aOne repetition of the exchange rotation protocol. After estimation of ΩLand ΩHas in Fig.3, the OPX adjusts exchange duration times\({\tilde{t}}_{l}\), using real-time knowledge of 〈ΩH〉, to rotate the qubit by user-defined target angles\({\theta }_{l}={\tilde{t}}_{l}\,\langle {{{\Omega }}}_{{{{{{{{\rm{H}}}}}}}}}\rangle\). Pulse durations\({\tilde{t}}_{\pi /2}\)for qubit initialization and readout use real-time knowledge of 〈ΩL〉.bEach row plots measurementsmjfrom one protocol repetition, hereM= 101 exchange probe outcomes.cEach row plots measurementmlfrom one protocol repetition, hereK= 101 controlled-exchange-rotation outcomes. To illustrate the increased coherence of controlled exchange rotations, we also plot in b and c the fraction of singlet outcomes of each column. 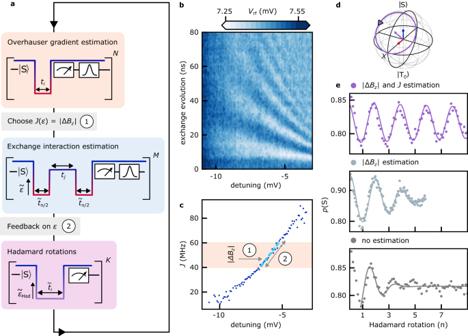Fig. 5: Real-time universal ST0control demonstrated by Hadamard rotations. aHadamard rotation protocol. After estimating ΩL,εis chosen in real-time such thatJ(ε) =∣ΔBz∣, based on a linearized offline model from panel c. If\(40\,{{{{{{{\rm{MHz}}}}}}}}\, < \,\left\langle | {{\Delta }}{B}_{z}| \right\rangle \, < \, 60\,{{{{{{{\rm{MHz}}}}}}}}\), the detuning is adjusted to account for deviations of the prevailingJfrom the offline model. Real-time knowledge of\({{{\Omega }}}_{{{{{{{{\rm{Had}}}}}}}}}=\sqrt{2}\,| {{\Delta }}{B}_{z}|\)then dictates\({\tilde{t}}_{i}\)to achieve a user-defined Hadamard rotation angle.bAveraged exchange driven FID as a function of detuning and evolution time. Here, a diabatic ΩL(π/2) pulse initializes the qubit near the equator of the Bloch sphere, prior to free exchange evolution, and subsequently prepares it for readout.cJas a function ofεextracted offline from b, as well as a linearized model (dashed line) used in the two feedback steps of panel a.dHadamard rotation depicted on the Bloch sphere.eMeasurement of Hadamard rotations with∣ΔBz∣andJestimation (purple, top panel), only∣ΔBz∣estimation (light gray, middle panel), and without the feedback shown in a (dark gray, bottom panel). Figure 4 a describes the real-time controlled exchange-driven rotations protocol aimed at stabilizing frequency fluctuations of the qubit at higher detunings. Following the approach of Fig. 3 , we first estimate Ω L and Ω H using real-time Bayesian estimation. We then use our knowledge of Ω H to increase the rotation angle coherence of the qubit where the exchange coupling is comparable with the Overhauser field gradient. Fig. 4: Real-time-controlled exchange-driven qubit rotations. a One repetition of the exchange rotation protocol. After estimation of Ω L and Ω H as in Fig. 3 , the OPX adjusts exchange duration times \({\tilde{t}}_{l}\) , using real-time knowledge of 〈Ω H 〉, to rotate the qubit by user-defined target angles \({\theta }_{l}={\tilde{t}}_{l}\,\langle {{{\Omega }}}_{{{{{{{{\rm{H}}}}}}}}}\rangle\) . Pulse durations \({\tilde{t}}_{\pi /2}\) for qubit initialization and readout use real-time knowledge of 〈Ω L 〉. b Each row plots measurements m j from one protocol repetition, here M = 101 exchange probe outcomes. c Each row plots measurement m l from one protocol repetition, here K = 101 controlled-exchange-rotation outcomes. To illustrate the increased coherence of controlled exchange rotations, we also plot in b and c the fraction of singlet outcomes of each column. Full size image As illustrated in Fig. 4 a, the qubit control pulses now respond in real time to both qubit frequencies Ω L and Ω H . Similar to the previous section, after determining 〈Ω L 〉 and confirming that 30 MHz < 〈Ω L 〉 < 50 MHz is fulfilled, the qubit is initialized near the equator of the Bloch sphere by fast diabatic Ω L ( π /2) pulses, followed by an exchange-based FID that probes Ω H . Based on the resulting 〈Ω H 〉, the OPX adjusts the separation times \({\tilde{t}}_{l}\) to rotate the qubit by user-defined target angles \({\theta }_{l}={\tilde{t}}_{l}\,\langle {{{\Omega }}}_{{{{{{{{\rm{H}}}}}}}}}\rangle\) . To show the resulting improvement of coherent exchange oscillations, we plot in Fig. 4 c the interleaved K = 101 measurements m l and compare them in Fig. 4 b to the M = 101 measurements m j . Fitting the average of the uncontrolled rotations by an oscillatory fit with Gaussian envelope decay yields \({T}_{{{{{{{{\rm{el}}}}}}}}}^{*}\,\approx\, 60\,{{{{{{{\rm{ns}}}}}}}}\) and Q ≈ 3, presumably limited by electrical noise [49] , while the quality factor of the controlled rotations is enhanced by a factor of two, Q ≈ 6. The online control of exchange-driven rotations using Bayesian inference stabilizes fluctuations of the qubit frequency at higher detunings, where fluctuations are more sensitive to detuning noise. Indeed, we attribute the slightly smaller quality factor, relative to Overhauser-driven rotations in Fig. 2 d, to an increased sensitivity to charge noise at larger detuning, which, owing to its high-frequency component, is more likely to fluctuate on the estimation timescales [36] . This section established for the first time stabilization of two rotation axes of a spin qubit. This advancement should allow for stabilized control over the entire Bloch sphere, which we demonstrate in the next section. Hadamard rotations In this experiment, we demonstrate universal ST 0 control that corrects for fluctuations in all Hamiltonian parameters. We execute controlled Hadamard rotations around \({\hat{{{{{{{{\boldsymbol{\omega }}}}}}}}}}_{{{{{{{{\rm{Had}}}}}}}}}\) , as depicted by the trajectory on the Bloch sphere of Fig. 5 d, by selecting the detuning ε Had in real time such that J ( ε Had ) = ∣ Δ B z ∣ . To achieve this, we do not assume that Δ B z = Ω L (i.e. we allow contributions of \({J}_{{{{{{{{\rm{res}}}}}}}}}\) to Ω L ) or that J = Ω L (i.e. we allow contributions of Δ B z to Ω H ). The full protocol is detailed in Supplementary Discussion . Fig. 5: Real-time universal ST 0 control demonstrated by Hadamard rotations. a Hadamard rotation protocol. After estimating Ω L , ε is chosen in real-time such that J ( ε ) = ∣ Δ B z ∣ , based on a linearized offline model from panel c. If \(40\,{{{{{{{\rm{MHz}}}}}}}}\, < \,\left\langle | {{\Delta }}{B}_{z}| \right\rangle \, < \, 60\,{{{{{{{\rm{MHz}}}}}}}}\) , the detuning is adjusted to account for deviations of the prevailing J from the offline model. Real-time knowledge of \({{{\Omega }}}_{{{{{{{{\rm{Had}}}}}}}}}=\sqrt{2}\,| {{\Delta }}{B}_{z}|\) then dictates \({\tilde{t}}_{i}\) to achieve a user-defined Hadamard rotation angle. b Averaged exchange driven FID as a function of detuning and evolution time. Here, a diabatic Ω L ( π /2) pulse initializes the qubit near the equator of the Bloch sphere, prior to free exchange evolution, and subsequently prepares it for readout. c J as a function of ε extracted offline from b, as well as a linearized model (dashed line) used in the two feedback steps of panel a. d Hadamard rotation depicted on the Bloch sphere. e Measurement of Hadamard rotations with ∣ Δ B z ∣ and J estimation (purple, top panel), only ∣ Δ B z ∣ estimation (light gray, middle panel), and without the feedback shown in a (dark gray, bottom panel). Full size image Real-time knowledge of both Δ B z and J would potentially benefit two-qubit gate fidelities [50] and the resonant-driving approach of previous works [35] , [38] , [39] . In the resonant implementation, constrained to the operating regime ∣ Δ B z ∣ ≫ J , low-frequency fluctuations of J result in transverse noise that causes dephasing and phase shifts of the Rabi rotations [51] , [52] . In previous sections, we have shown how to probe the qubit Larmor frequencies Ω H and Ω L at different detunings in real time and correct for their fluctuations. Now, we simultaneously counteract fluctuations in J and ∣ Δ B z ∣ on the OPX in order to perform the Hadamard gate. As we do not measure the sign of Δ B z , we identify the polar angle of \({\hat{{{{{{{{\boldsymbol{\omega }}}}}}}}}}_{{{{{{{{\rm{Had}}}}}}}}}\) as either φ = π /4 or − π /4. In other words, starting from the singlet state, the qubit rotates towards + X on the Bloch sphere for one sign of Δ B z , and towards − X for the other sign. The sign of the gradient may change over long time scales due to nuclear spin diffusion (on the order of many seconds [41] ), but the measurement outcomes of our protocol are expected to be independent of the sign. The relative sign of Overhauser gradients becomes relevant for multi-qubit experiments [53] , and could be determined [54] by comparing the relaxation time of the ground state (e.g. \(| \uparrow \downarrow\, \rangle\) ) of Δ B z with its excited state ( \(| \downarrow \uparrow \,\rangle\) ). Such diagnostic sign-probing cycles on the FPGA should not require more than a few milliseconds, negligible compared to the expected time between sign reversals. In preparation for our protocol, we first extract the time-averaged exchange profile by performing exchange oscillations as a function of evolution time [Fig. 5 b]. Removing contributions of Δ B z to Ω H then yields J ( ε ) in Fig. 5 c. A linear approximation in the target range 40 MHz < 〈 J 〉 < 60 MHz (dashed blue line) is needed later on the OPX to allow initial detuning guesses when tuning up J ( ε ) = ∣ Δ B z ∣ . We also provide the OPX with a value for the residual exchange at low detuning, \({J}_{{{{{{{{\rm{res}}}}}}}}}\,\approx \,20\,{{{{{{{\rm{MHz}}}}}}}}\) , determined offline as described in Supplementary Fig. 5 . As illustrated in Fig. 5 a, the Hadamard rotation protocol starts by estimating ∣ Δ B z ∣ from Ω L , taking into account a constant residual exchange by solving \({{\Delta }}{B}_{z}^{2}={{{\Omega }}}_{{{{{{{{\rm{L}}}}}}}}}^{2}-{J}_{{{{{{{{\rm{res}}}}}}}}}^{2}\) . Next, an initial value of ε Had is chosen based on the linear offline model to fulfill J ( ε Had ) = ∣ Δ B z ∣ [feedback in panel (a,c)]. To detect any deviations of the prevailing J from the offline model, an exchange-driven FID is performed at ε Had to estimate J from Ω H , using \({J}^{2}={{{\Omega }}}_{{{{{{{{\rm{H}}}}}}}}}^{2}-{{\Delta }}{B}_{z}^{2}\) . Any deviation of 〈 J 〉 from the target value ∣ Δ B z ∣ is subsequently corrected for by updating ε Had based on the linearized J ( ε ) model [feedback in panels (a,c)]. Matching J to ∣ Δ B z ∣ in the two detuning feedback steps each takes about 400 ns on the OPX. Finally, real-time knowledge of \({{{\Omega }}}_{{{{{{{{\rm{Had}}}}}}}}}\equiv \sqrt{2}| {{\Delta }}{B}_{z}|\) is used to generate the free evolution times \({\tilde{t}}_{i}\) , spent at the updated value \({\tilde{\varepsilon }}_{{{{{{{{\rm{Had}}}}}}}}}\) , in order to perform Hadamard rotations by K user defined target angles. The resulting Hadamard oscillations are shown in Fig. 5 e (top panel) and fitted with an exponentially decaying sinusoid, indicating a quality factor Q > 5. (According to this naive fit, the amplitude drops to 1/e over approximately 40 rotations, although we have not experimentally explored rotation angles beyond 9 π .) In comparison to exchange-controlled rotations from Fig. 4 c, the Hadamard rotations are more stable, which we attribute to the additional feedback on detuning that fixes the oscillation axis and decreases sensitivity to charge noise. To illustrate the crucial role of real-time estimation for this experiment, we also performed rotation experiments that do not involve any real-time estimation and feedback cycles (dark gray data, bottom panel), as follows. Within minutes after performing the controlled Hadamard rotations (purple data), we executed Hadamard rotations assuming a fixed value of \(| {{\Delta }}{B}_{z}|=\overline{| {{\Delta }}{B}_{z}| }\) , i.e. by pulsing to a fixed detuning value corresponding to \(J({\varepsilon }_{{{{{{{{\rm{H}}}}}}}}})=\overline{| {{\Delta }}{B}_{z}| }\) according to the offline model. Here, \(\overline{| {{\Delta }}{B}_{z}| }\approx 40\) MHz is the average Overhauser gradient that we observed just before executing the Hadamard protocol. Not surprisingly, the quality factor of the resulting Hadamard-like oscillations is low and the rotation angle deviates from the intended target angle, likely due to the Overhauser gradient having drifted in time. As a side note, we mention that the purple data in Fig. 5 e constitutes an average over 5000 repetitions, corresponding to a total acquisition time of 2 minutes including Overhauser and exchange estimation cycles. In contrast, the dark gray data also constitutes an average over 5000 repetitions, but only required 15 seconds because of the omission of all estimation and feedback cycles. To verify that the enhancement in Q is not solely due to the more accurate knowledge of ∣ Δ B z ∣ , we also performed Hadamard rotations only using the estimation of ∣ Δ B z ∣ . The FPGA was programmed to perform a measurement where the initialized singlet is pulsed to a fixed detuning J ( ε H ) ≈ 20 MHz to perform a Hadamard rotation, only if the estimated ∣ Δ B z ∣ on the FPGA satisfies \(17\,{{{{{{{\rm{MHz}}}}}}}}\, < \,\left\langle | {{\Delta }}{B}_{z}| \right\rangle \, < \,23\,{{{{{{{\rm{MHz}}}}}}}}\) . We then post select the repetitions where \(19.5\,{{{{{{{\rm{MHz}}}}}}}}\, < \,\left\langle | {{\Delta }}{B}_{z}| \right\rangle \, < \, 20.5\,{{{{{{{\rm{MHz}}}}}}}}\) . Fitting this by an oscillatory fit with Gaussian envelope decay yields \({T}_{{{{{{{{\rm{el}}}}}}}}}^{*}\,\approx\, 70\,{{{{{{{\rm{ns}}}}}}}}\) , Q ≈ 2.0 and frequency ≈ 29 MHz. In Fig. 5 e we compare these data (light gray, middle panel) with the cases where the FPGA estimated both ∣ Δ B z ∣ and J (purple, top panel) and where the microprocessor does not perform any estimation but simply pulses to J ( ε H ) to perform the rotations (dark gray, bottom panel). (In the middle panel the horizontal axis was rescaled to the Hadamard evolution time using the fitted frequency ≈ 29 MHz.) We see that (i) a reduction of the uncertainty in ∣ Δ B z ∣ from ≈ 30 MHz (r.m.s.) to ≈ 2 MHz (dark gray to light gray) does not yield a proportional gain in Q and (ii) the improvement in Q when including estimation of J (light gray to purple) is much larger than can be justified solely by the slight further reduction of the uncertainty in ∣ Δ B z ∣ (roughly from ≈ 2 MHz to ≈ 1 MHz). This demonstrates the crucial contribution of the estimations along both axes in the improvement of our Hadamard gate quality factor. Further evidence for the fluctuating nature of non-stabilized Hadamard rotations is discussed in Supplementary Fig. 6 . The stabilized Hadamard rotations demonstrate real-time feedback control based on Bayesian estimation of J and ∣ Δ B z ∣ , and suggest a significant improvement in coherence for ST 0 qubit rotations around a tilted control axis. Despite the presence of fluctuations in all Hamiltonian parameters, we report effectively constant amplitude of Hadamard oscillations, with a reduced visibility that we tentatively attribute to estimation and readout errors. Our experiments demonstrate the effectiveness of feedback control in stabilizing and improving the performance of a singlet-triplet spin qubit. The protocols presented showcase two-axis control of a qubit with two fluctuating Hamiltonian parameters, made possible by implementing online Bayesian estimation and feedback on a low-latency FPGA-powered qubit control system. Real-time estimation allows control pulses to counteract fluctuations in the Overhauser gradient, enabling controlled Overhauser-driven rotations without the need for micromagnets or nuclear polarization protocols. Notably, even in the absence of a deterministic component of the Hamiltonian purely noise-driven coherent rotations of a two-level quantum system were demonstrated. The approach is extended to the real-time estimation of the second rotation axis, dominated by exchange interaction, which we then combine with an adaptive feedback loop to generate and stabilize Hadamard rotations. In particular, executing the Hadamard gate involves (i) sequentially executing two distinct estimation cycles, where the design of the second cycle relies on the outcomes of the first, (ii) correlating the detected frequencies to distinguish independent fluctuations of the two control axes, and (iii) utilizing this correlated information to dynamically construct and execute a Hadamard gate. These steps demand real-time adaptive estimations and signal generations throughout the protocol, which has not been demonstrated before. A constant Overhauser field gradient, whether stemming from nuclear spin pumping or a micromagnet, is expected to further improve the feedback control. From this perspective, our work represents a worst-case scenario, demonstrating the effectiveness of our experimental technique. Our protocols assume that Δ B z does not depend on the precise dot detuning in the (1,1) configuration and remains constant on the time scale of one estimation. Similarly, stabilization of exchange rotations is only effective for electrical fluctuations that are slow compared to one estimation. Therefore, we expect potential for further improvements by more efficient estimation methods, for example through adaptive schemes [55] for Bayesian estimation from fewer samples, or by taking into account the statistical properties of a time-varying signal described by a Wiener process [56] or a nuclear spin bath [57] . Machine learning could be used to predict the qubit dynamics [58] , [59] , [60] , possibly via long short-term memory artificial neural networks as reported for superconducting qubits [61] . While our current qubit cycle time (approximately 30 μs) is dominated by readout and qubit initialization, it can potentially be reduced to a few microseconds through faster qubit state classification, such as enhanced latched readout [48] , and faster reset, such as fast exchange of one electron with the reservoir [62] . Our protocol could be modified for real-time non-local noise correlations [63] or in-situ qubit tomography using fast Bayesian tomography [64] to study the underlying physics of the noisy environment, thereby providing qualitatively new insights into processes affecting qubit coherence and multi-qubit error correction. Beyond ST 0 qubits, our protocols uncover new perspectives on coherent control of quantum systems manipulated by baseband pulses. This work represents a significant advancement in quantum control by implementing an FPGA-powered technique to stabilize in real time the qubit frequency at different manipulation points. Experimental setup We use an Oxford Instruments Triton 200 cryofree dilution refrigerator with base temperature below 30 mK. The experimental setup employs a Quantum Machines OPX+ for radio-frequency (RF) reflectometry and gate control pulses. The RF carrier frequency is ≈158 MHz and the gate control pulses sent to the left and right plunger gates of the DQD are filtered with low-pass filters (≈220 MHz) at room temperature, before being attenuated at different stages of the refrigerator. Low-frequency tuning voltages (high-frequency baseband waveforms) are applied by a QDAC [65] (OPX) via a QBoard high-bandwidth sample holder [66] . Measurement details Before qubit manipulation, an additional reflectometry measurement is taken as a reference to counteract slow drifts in the sensor dot signal. At the end of each qubit cycle, a ≈ 1 μs long pulse is applied to discharge the bias tee. As the qubit cycle period (tens of μs) is much shorter than the bias tee cutoff (≈300 Hz), we do not correct the pulses for the transfer function of the bias tee.